Realistic loophole-free Bell test with atom–photon entanglement The establishment of nonlocal correlations, guaranteed through the violation of a Bell inequality, is not only important from a fundamental point of view but constitutes the basis for device-independent quantum information technologies. Although several nonlocality tests have been conducted so far, all of them suffered from either locality or detection loopholes. Among the proposals for overcoming these problems are the use of atom–photon entanglement and hybrid photonic measurements (for example, photodetection and homodyning). Recent studies have suggested that the use of atom–photon entanglement can lead to Bell inequality violations with moderate transmission and detection efficiencies. Here we combine these ideas and propose an experimental setup realizing a simple atom–photon entangled state that can be used to obtain nonlocality when considering realistic experimental parameters including detection efficiencies and losses due to required propagation distances. In recent years, several applications of quantum nonlocality have been proposed [1] , [2] , [3] , [4] (see a recent review on Bell nonlocality [5] ). These proposals are based on the fact that nonlocal correlations can be certified without any assumption on the internal mechanisms of the devices used in the experiment. Thus, once established, nonlocal correlations can be used in what is now referred to as device-independent protocols. Nonlocal correlations can be obtained by measuring entangled quantum systems in appropriately chosen local observables. This is called a Bell test as the nonlocal nature of the measurement outcomes can be certified by the violation of certain constraints known as Bell inequalities [5] . Many Bell tests have been conducted in the last few decades, but no nonlocal correlations have been strictly established so far. This is because all of the performed experiments suffered either from the detection loophole or from the locality loophole [5] . Experiments using entangled photons have reported Bell inequality violations closing the locality [6] , [7] , [8] and detection [9] loopholes separately. On the other hand, the detection loophole has been closed with stationary systems like atoms, ions and circuits [10] , [11] , [12] . The main technological challenge to closing both loopholes simultaneously is having both efficient detection and long-distance entanglement. In this work, we propose an experimental setup involving available technology to implement a loophole-free Bell test. It uses a single atom coupled to the field of a cavity in order to produce a specific entangled state between the atom and the light emitted by the cavity and combines efficient detection schemes on the atomic side and the coherent nature of the light field to perform hybrid detection on the photonic side [13] , [14] . Our scheme considers the experimental effects neglected in previous proposals [15] , [16] and thus positions current atom–photon systems as good candidates for demonstrating loophole-free nonlocal correlations. The paper is structured as follows: first, we introduce the target state and the measurement settings used in the Bell test. We then give an explanation on how this state can be produced by means of cavity quantum electrodynamics (QED) techniques and discuss the relevant and feasible parameter regime that yields the desired state. We also discuss an implementation of our scheme in optical cavities and optimize the Clauser–Horne–Shimony–Holt (CHSH) inequality [17] violation for currently available experimental parameters. Finally, we discuss possible circuit QED implementations in the final section and compare our proposal with previous ones. The ideal case Our proposal takes advantage of two facts first noticed in Brunner et al . [18] and Cabello and Larsson [19] . First, highly efficient detections are typically available for the electronic levels of single atoms [20] . At the same time, photons propagating either in free space or in low-loss optical fibres are excellent candidates for carriers of information over long distances. Further, the combination of highly efficient homodyne detection with photodetection greatly reduces the required minimum photodetection efficiency [13] , [14] , [15] , [16] , [21] . Our starting point is to consider a state of the form where and are two atomic states and and denote states of the electromagnetic field (vacuum and a coherent state, respectively) with where is the n th energy eigenstate of the field. As will be described below, this state violates a Bell inequality even for low-efficiency photodetection and can be well approximated with current technology. Although we motivated this work by considering a real atom, the state (1) can, in principle, be devised using different platforms—for example, superconducting qubits, quantum dots, nitrogen-vacancy centres and equivalent systems. We consider the CHSH Bell inequality [17] , which states that the correlations obtained are nonlocal if the following inequality is violated: where ρ is the quantum state under scrutiny and denotes the Bell operator with A i and B j being observables with outcomes ±1. Here we set the atomic observables as where σ i is the usual Pauli matrix. In the photonic part, we consider dichotomized photodetection and X quadrature operators with binning b (homodyne detection) [13] , [14] : where is the eigenstate of the quadrature operator , and a is the annihilation operator of the field. As quadrature measurements can be made very efficient (nearly perfect), there will be an asymmetry in the total efficiency of the photonic measurements: the total homodyning efficiency will be basically determined by transmission losses, whereas the total photodetection efficiency will be composed of transmission and typical photodetector efficiency. We thus model the transmission losses with a beam splitter with transmittance t line (affecting both the photodetector and the homodyning apparatus) and the photodetector intrinsic efficiency as a beam splitter with transmittance followed by a perfect detector. 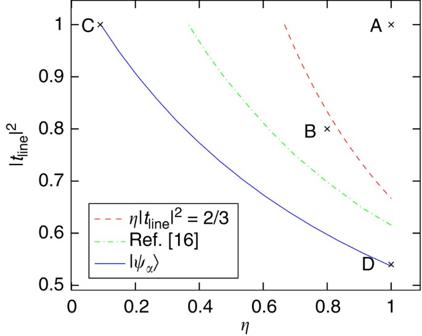Figure 1: Critical line above which CHSH violations are obtained. The blue line corresponds to the ideal state of our proposal. The parametersα, γ, vandbwere optimized for each point. For comparison, we include the curveη|tline|2=2/3 (red) that results from the Eberhard bound22,23, and the curve from the best experimental proposal to date in Sangouardet al.16(green). For the sake of illustration, we give the specific numbers for the points represented by crosses A, B, C and D inTable 1. Figure 1 summarizes the results. In ideal conditions (that is, point A in Table 1 ), the CHSH value can reach =2.32 for | α |=2.1, which translates into an average of 4.41 photons in the coherent state. Moreover, a violation can be found even for η =0.15 with | t line | 2 =1 (point C in Table 1 ), or for transmittance | t line | 2 =0.55 with η =1 (point D in Table 1 ). Also, for a detection efficiency of η =0.8 and a transmission of | t line | 2 =0.8 we find a CHSH value of 2.07 (point B in Table 1 ). For comparison, we have also included the curve η | t line | 2 =2/3 that results from the Eberhard bound [22] , [23] , which is the required efficiency and transmission to perform a loophole-free experiment with photon polarization, and the curve from the best experimental proposal to date involving an atom and a photonic mode [16] . Figure 1: Critical line above which CHSH violations are obtained. The blue line corresponds to the ideal state of our proposal. The parameters α, γ, v and b were optimized for each point. For comparison, we include the curve η | t line | 2 =2/3 (red) that results from the Eberhard bound [22] , [23] , and the curve from the best experimental proposal to date in Sangouard et al . [16] (green). For the sake of illustration, we give the specific numbers for the points represented by crosses A, B, C and D in Table 1 . Full size image Table 1 Optimized parameters for four points on Fig. 1. Full size table Realistic scenario We now show a scheme aiming to produce the state (1) in a cavity QED scenario. The first part of the scheme is depicted in Fig. 2a . An input field is incident on a cavity with a single three-level atom prepared initially in a superposition of the states g and s : . 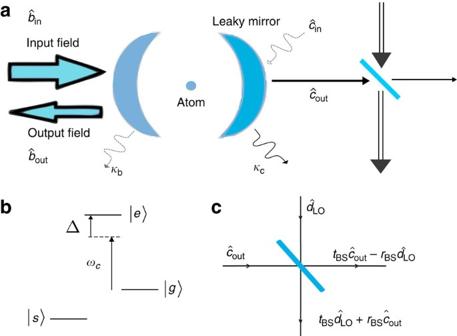Figure 2: State preparation. (a) An input field is incident on a cavity with an atom in the dispersive regime. This causes some reflection and some transmission of the cavity field. We assume that the mirror on the right has a lower reflectivity than the mirror on the left, such that the field predominantly leaves the cavity to the right. The final beam splitter performs a displacement operation, which creates a superposition of propagating vacuum and coherent state. (b) Level structure of the atom. The cavity field is dispersively coupled to thetransition, and thestate is assumed to be far detuned such that it does not interact with the cavity field. (c) Beam splitter convention used. A displacement operation is applied on the mode labelledĉoutby combining it with a local oscillator (mode labelled). Figure 2b shows the level structure of the atom. Transition is coupled dispersively to the cavity with detuning Δ= ω ge − ω c , where ω c is the cavity frequency and ω ge is the frequency of the transition . The cavity is asymmetric with decay rates of the mirrors κ b << κ c and a cavity decay rate κ=κ b + κ c . This means that the field leaks out of the cavity essentially only through the right mirror (cf. Fig. 2a ). The fact that one needs an asymmetric cavity is not a priori obvious and will be explained below. We assume that the level is detuned far enough such that it does not interact with the cavity field. Figure 2: State preparation. ( a ) An input field is incident on a cavity with an atom in the dispersive regime. This causes some reflection and some transmission of the cavity field. We assume that the mirror on the right has a lower reflectivity than the mirror on the left, such that the field predominantly leaves the cavity to the right. The final beam splitter performs a displacement operation, which creates a superposition of propagating vacuum and coherent state. ( b ) Level structure of the atom. The cavity field is dispersively coupled to the transition, and the state is assumed to be far detuned such that it does not interact with the cavity field. ( c ) Beam splitter convention used. A displacement operation is applied on the mode labelled ĉ out by combining it with a local oscillator (mode labelled ). Full size image As the cavity transmission depends on the atomic state, the atom–cavity system acts as a filter that transforms the initial state in the following way: where and represent the reflected and transmitted photonic states, α in is the complex amplitude of the input coherent state and r j and t j ( j = s , g ) are the amplitude reflectivity and transmitivity of the empty cavity (atom in the state , that is, j = s ) and of the cavity with the atom (atom in the state , that is, j = g ) and | r j | 2 +| t j | 2 =1. Notice that we assume that both the reflected and transmitted fields are still coherent states (see Methods for details). In order to produce a state of the form (1), one needs to meet the following conditions: t s =0 with and , where is the desired coherent state in (1). An alternative is to apply a displacement on the transmitted field [24] . The displacement is just the result of combining a field exiting the atom–cavity system ( ĉ out mode) with a coherent local oscillator ( mode) on a beam splitter, as depicted in Fig. 2c . The output port of interest is the port with the output field , where r BS and t BS are the amplitude reflectivity and transmitivity of the beam splitter, respectively. For a coherent state, , in the ĉ out mode, one can achieve a zero amplitude in this output port by tuning the amplitude of such that r BS β = t BS α x . In our case, α x = t s α in , and one can obtain the state contained in (1). The full Bell test setup is shown in Fig. 3 . The beam splitters are identical with the property | t BS | 2 >>| r BS | 2 . Note that, in order to satisfy the condition r BS β = t BS α x , the spatiotemporal modes of the two coherent states α x and β must be identical. This can be achieved, for example, by using an auxiliary cavity similar to the one containing the atom (see Fig. 3 ), where α x = t s α in . Eventually, instead of using the auxiliary cavity, one might look for an atom–cavity–laser configuration in which the coupling of the field of polarization connecting the state with some excited state is negligible compared with the dispersive coupling of the transition, and the orthogonal polarization couples to neither , nor . In such a situation, one might use this field to produce the displacement pulse using only a single cavity. 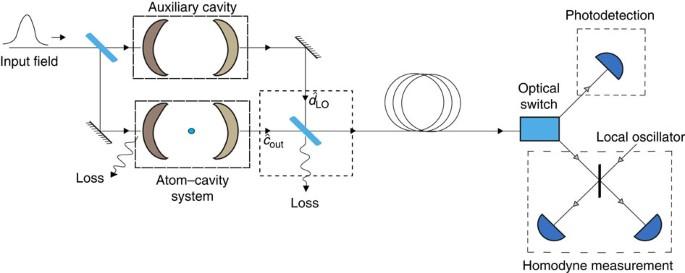Figure 3: Possible experimental setup. A pulse of light is first split on a beam splitter (blue). Part of it goes to the atom–cavity system (lower branch) described inFig. 2. The other part of the split pulse passes through an auxiliary cavity (upper branch), which is used to produce a pulse with the same spectral properties as that produced when the atom is in thestate. This requirement has to be met for a perfect displacement in the second beam splitter. Both beam splitters have the property that |tBS|2>>|rBS|2. After the state preparation, the photonic part of the state goes to a location that, given the times necessary for choosing the measurement and registering the results, assures space-like separation, and is submitted to either photodetection or homodyne measurement. (Possible detection schemes of the atomic state are explained in the text). Figure 3: Possible experimental setup. A pulse of light is first split on a beam splitter (blue). Part of it goes to the atom–cavity system (lower branch) described in Fig. 2 . The other part of the split pulse passes through an auxiliary cavity (upper branch), which is used to produce a pulse with the same spectral properties as that produced when the atom is in the state. This requirement has to be met for a perfect displacement in the second beam splitter. Both beam splitters have the property that | t BS | 2 >>| r BS | 2 . After the state preparation, the photonic part of the state goes to a location that, given the times necessary for choosing the measurement and registering the results, assures space-like separation, and is submitted to either photodetection or homodyne measurement. (Possible detection schemes of the atomic state are explained in the text). Full size image The problem of an input coherent pulse with frequency spectrum s L ( ω ) and amplitude α in impinging on an atom–cavity system can be treated using input–output theory [25] (see Methods for details). This gives the form of the atomic state-dependent amplitude reflection and transmission coefficients, r j ( ω ) and t j ( ω ), j = s , g as functions of the input pulse. The final atom-field state is obtained upon tracing away non-radiative losses in the cavity mirrors, the fields reflected by the cavity, emitted by the atom and the other output port of the beam splitter. This naturally leads to coherence (and entanglement) loss and results, when the atom is initially prepared in the state , in the mixed state where and the visibility V is (see Methods for details), where C is the usual single-atom cooperativity and is a factor that describes the asymmetry of the cavity. Here the continuous frequency coherent state, , is with the transmission coefficients and the atomic state is initially prepared with φ (see paragraph before equation (9)) such that the final state is of the form (10). In the above, s L ( ω ) is the frequency spectrum of the laser field, g is the coupling constant of the cavity mode to the transition, Г is the transverse decay rate of the state and κ L is the loss rate of the cavity mirrors. From equation (12), it is easy to see that, for F →0, we have V →1. Also for F →0, we need the three conditions, r BS →0, f cav →0 and C →∞. In practice, the first condition means that one should use a small value of the beam splitter reflectivity and adjust the amplitude of the local oscillator, such that the condition r BS β = t BS t s α in is still satisfied. The second condition is precisely the requirement of the asymmetric cavity we have mentioned at the beginning of this section and is dependent only on the transmission and losses of the cavity mirrors. For completeness, we have also included non-radiative mirror losses. The third condition means that one needs large single-atom cooperativity. One remarkable feature of this result is that, for C >>1, the visibility V (but of course not the state) is independent of the details of the spectrum of the input pulse. The final point to note is that, to satisfy the approximations used in our derivation, we require a negligible probability of exciting the atom throughout the duration of the input pulse. This is important, as, to maintain some specific amplitude of the output coherent state after the beam splitter, one might have to use a very large amplitude input laser if the integral in equation (17) is small. For the sake of this theoretical analysis, we consider the case of an input Gaussian pulse with the normalized spectrum where ω L is the central laser frequency, and γ L is the bandwidth of the pulse. To close the locality loophole, one has to propagate the outgoing pulse for some minimum distance, given by the larger of the measurement times of the atom and the pulse, which depends on the pulse duration. The pulse duration is given by the relevant time scale of the system—that is, either by the input pulse duration or by the cavity lifetime, whichever is greater. This means that, from the point of view of closing the locality loophole, it is useful to push the duration of the input pulse down to the cavity lifetime, but not necessarily further. As the pulse duration and the cavity lifetime are proportional to the inverse of the pulse bandwidth γ L and the cavity decay rate κ , respectively, the best case would be if γ L ≈ κ . 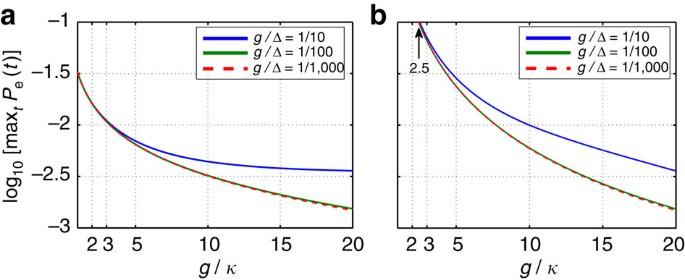Figure 4: Log plots of the maximum probability of atomic excitation. This figure shows plots of log10[maxtPe(t)] as a function of the parameterg/κ, assuming that the central laser frequency is on resonance with the bare cavity, for different values ofg/Δ. (a) The case with input pulse with minimal bandwidth settingg/γL=max(g/κ). (b) The case with input pulse bandwidth set equal to the cavity bandwidth (g/γL=g/κ). Forg/Δ small enough, the probability of exciting the atom becomes insensitive to the precise value ofg/Δ. This fact is illustrated by the overlap of curves corresponding tog/Δ=1/100 andg/Δ=1/1,000. The parameters used in this plot are |α|=2.1,fcav=4/100 andg/Г=5/3. Figure 4 shows plots of log 10 [max t P e ( t )], the maximum probability of exciting the atom as a function of the parameter g / κ (the coupling strength over the total cavity decay rate), assuming that the central laser frequency is on resonance with the bare cavity, for g /Δ=1/10, 1/100, 1/1,000. Figure 4a is the case for a fixed minimal bandwidth of the input pulse, in the sense that we choose γ L such that g / γ L =max( g / κ ). Figure 4b corresponds to the situation when the input pulse bandwidth is set equal to the cavity bandwidth in order to minimize the pulse duration. In the following, we will consider the regions where (max t P e ( t ))≤0.1 as the parameter regimes for which our analysis is suitable. As is evident from Fig. 4 , for some large g / γ L values, there always exist some g / κ values for which our solutions are self-consistent, which is not the case when γ L = κ , the situation minimizing the pulse duration. We can thus look for some intermediate value of γ L (having all the other parameters fixed), which minimizes the pulse duration while still respecting the validity of the used approximation. This is the strategy we employ in the next section, in which we will discuss a possible implementation of our scheme using realistic experimental parameters. Figure 4: Log plots of the maximum probability of atomic excitation. This figure shows plots of log 10 [max t P e ( t )] as a function of the parameter g / κ , assuming that the central laser frequency is on resonance with the bare cavity, for different values of g /Δ. ( a ) The case with input pulse with minimal bandwidth setting g / γ L =max( g / κ ). ( b ) The case with input pulse bandwidth set equal to the cavity bandwidth ( g / γ L = g / κ ). For g /Δ small enough, the probability of exciting the atom becomes insensitive to the precise value of g /Δ. This fact is illustrated by the overlap of curves corresponding to g /Δ=1/100 and g /Δ=1/1,000. The parameters used in this plot are | α |=2.1, f cav =4/100 and g /Г=5/3. Full size image Experimental feasibility So far, we have theoretically described a general cavity scenario. In the following, we will focus our attention on possible implementations of our scheme in optical cavities. This implementation has the advantage of allowing large propagation distances due to the availability of low-loss optical fibres. We start by general constraints on measurement times and propagation distances imposed by the locality loophole. To close the locality loophole, one requires the start of the measurement event on one side to be space-like separated from the end of the measurement event on the other side. In other words, we need that the space–time coordinates of the end of the atomic measurement and the choice of measurement basis (photon detection or homodyning) on the photonic side be space-like separated, and vice versa. This constraint translates into the minimum propagation distance where c is the speed of light in free space; Δ t at/ph,c is the time required on the atomic/photonic side to choose the measurement settings, which also includes the time to change the measurement basis; and Δ t at/ph,m is the time required on the atomic/photonic side to perform the actual measurement, which necessarily includes the duration of the light pulse. We assume that the main time constraint is set by the atomic measurement, which is typically slower than the measurement of photons. The above equation shows that, even if we used a very short pulse, we would still need to propagate it at least to a distance, which is given by the sum of atomic measurement time and the time required to choose a basis (a rotation in the space of and , typically using RF pulses), multiplied by c . The best trade-off in this case is thus to have Δ t ph,m ≈Δ t at,m +Δ t at,c . This is possible because the time needed to choose a basis on the photonic side can be very fast [7] . One possible way for performing a fast atomic state detection would be the use of a two-photon ionization technique [20] . This technique has been performed in free-space configurations and can achieve 98% efficiency in <1 μs. Although the restriction of a small cavity might make such a photoionization technique technically challenging, proposals to make focusing cavities with large physical volumes (lengths of ~1 cm) while still maintaining large coupling constants ( g ~100 MHz) exist [26] , [27] , potentially making such techniques compatible. Here we assume Δ t at,m +Δ t at,c =1 μs. We should thus seek to produce a pulse that requires a total measurement duration of up to 1 μs. For the Gaussian pulse example considered in our calculation, we take the total pulse measurement duration to be Δ t ph,m =6 / γ L,m . The factor 6 is chosen such that if the bandwidth of the pulse incident on the cavity is γ L,m , then the neglected tails of the outgoing pulse correspond to <0.5% of the total integrated intensity of the outgoing pulse (for the parameters used in Table 2 , see below). For a measurement time of 1 μs, this corresponds to γ L,m =2 π × 1.35 MHz. It also means that, for outgoing pulse bandwidths γ L > γ L,m (shorter pulses), the total measurement time is set by Δ t at,m +Δ t at,c =1 μs and the minimum propagation distance is 300 m. Table 2 Derived visibilities with available experimental parameters Full size table Next, we use experimental parameters given in [28] , [29] , [30] . These experiments use 852 and 780 nm light, respectively, which are subject to about 2 dB km −1 loss in optical fibres. In the following, we compare both experiments and possible modifications. As discussed previously, we will work in the large detuning regime, Δ>> g . We choose an arbitrary, but subjected to experimental constraints, value of g /Δ=1/10. This ensures that we respect all approximations used, as long as we also satisfy the condition max t P e ( t )≤0.1. The figures of merit in both cases will be γ 0.1 , which is the largest acceptable laser bandwidth that satisfies condition max t P e ( t )≈0.1, and the state production visibility (12), which is computed using the actual laser bandwidth ≡min( κ , γ 0.1 , γ L,m ). We also include the effect of finite pulse measurement time on the visibility, using (12)–(15). We assume | α |=2.1 and | r BS | 2 =0.001. Table 2 summarizes the results. The parameters mentioned by Birnbaum et al . [28] and Hood [29] are ( g /(2 π ), κ /(2 π ), Г/(2 π ), f cav )=(34, 4.1, 2.6 MHz, 10/4) (we assume that the experiment performed implements a symmetric cavity). Owing to the symmetry of the cavity, one obtains a small effective visibility. Assuming that the cavity could be made asymmetric by reducing f cav to the current value in the experiment by Ritter et al . [30] , the visibility markedly increases to 72.7% (second row). Neglecting the mirror losses, we show in the third row that V can be as high as 90.8%. The parameters used by Ritter et al . [30] are ( g /(2 π ), κ /(2 π ), Г/(2 π ), f cav )=(5, 3 and 3 MHz, 14/100). As the setup stands, the visibility is 56.3%. However, neglecting the mirror losses, V increases to 71.3% (fifth row). If it were further possible to reduce the total cavity decay rate by a factor of 2, thus increasing the cooperativity, while maintaining the same asymmetry, the visibility further increases to 77.2% (sixth row). The required incident photon number can be calculated from (17). For the parameters in Table 2 and requiring the resulting photon number, =4.41, one requires | α in | 2 ≈25–400 input photons. For the specific case of 87 Rb, one might also identify possible states playing the role of , and . We may choose, for example, the state to be the hyperfine state , the state to be and the state to be . In this case, the input pulse and cavity field would have a σ + polarization coupling the transition. Owing to the large detuning of the hyperfine states (6.8 GHz), and the fact that the s state is far detuned to any other σ + transitions, these states are possible candidates for the experiment. We now maximize as a function of transmission and detector inefficiency for a set of realistic parameters. We thus set | α |=2.1, ( g /(2 π ), κ /(2 π ), Г/(2 π ), f cav )=(34, 4.1 and 2.6 MHz, 14/100) and | r BS | 2 =0.001 (second row of Table 2 ). Notice that we have included possible non-radiative losses from cavity mirrors. Given these constraints, the maximal CHSH violation is 2.17. Moreover, we can attain a violation even for η =0.37 with | t line | 2 =1, or transmittance | t line | 2 =0.68 with η =1. 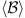Figure 5: Contour lines ofas a function ofηand |tline|2. In this plot, we fixed |α|=2.1 and optimized the measurement and state parametersγ, bandvfor each point. The parameters used are (g/(2π),κ/(2π), Г/(2π),fcav)=(34, 4.1 and 2.6 MHz, 14/100) and |rBS|2=0.001 (second row ofTable 2). The result for the ideal state in (1) (dotted line) is included for comparison. For the sake of illustration we give the specific numbers for the points represented by crosses A, B and C inTable 3. Figure 5 summarizes these results. Note that the higher the visibility of the produced state, the closer one gets to the ideal scenario (dashed line in Fig. 5 ). Figure 5: Contour lines of as a function of η and | t line | 2 . In this plot, we fixed | α |=2.1 and optimized the measurement and state parameters γ, b and v for each point. The parameters used are ( g /(2 π ), κ /(2 π ), Г/(2 π ), f cav )=(34, 4.1 and 2.6 MHz, 14/100) and | r BS | 2 =0.001 (second row of Table 2 ). The result for the ideal state in (1) (dotted line) is included for comparison. For the sake of illustration we give the specific numbers for the points represented by crosses A, B and C in Table 3 . Full size image In this work, we have shown that using current technology it is possible to produce a hybrid atom–photon entangled state that still violates the CHSH inequality up to a value of 2.17. We also showed that we can attain a violation even for a low photon counting efficiency of 37% with perfect transmission, or a line transmission of 68% with perfect detection efficiency. Moreover, assuming that it is possible to perform photoionization measurements <1 μs, the required propagation distances to close the locality loophole are of the order of 300 m for optical setups. This gives a very good outlook for optical systems in eventually performing a loophole-free Bell test. In principle, one may also consider circuit QED setups. The advantages of such setups are twofold. First, the very fast and efficient qubit state detection, on the order of 10 ns [12] , potentially lowers the required propagation distances to laboratory-scale distances (10 m or less). Second, in this system, large ratios of coupling constant to cavity decay, g / κ , can be achieved. The drawbacks with current technology are the limited efficiencies of both photodetection and homodyne detection (private communication with Steve Girvin) and the requirement to cool the propagation line down to cryogenic temperatures. The hope is that both these drawbacks, being of technological nature, can be eventually overcome in near-future experiments. Before concluding, let us compare our present results with previous proposals involving similar setups. In the study by Sangouard et al . [16] , a Bell test involving the production of an entangled state between an atom and a photonic field created by atomic decay was studied (see also Brask and Chaves [31] ). It was shown that Bell violations with photodetection efficiency of 39% (see green curve in Fig. 1 ) can be achieved. Note, however, that this number refers to the ideal state, considering that all light emitted by the atom is collected. Our scheme overcomes this problem as the photonic part of the state is the transmitted mode and, moreover, requires lower efficiencies. We believe that our proposal will trigger possible implementations of loophole-free Bell tests with atom–photon interfaces, which are particularly important in quantum communication and cryptographic applications. Input–output relations Here we derive the input–output relations [25] for a two-sided cavity, clearly stating the approximations used and their validity. We consider a cavity mode ( a mode) that couples to a left mode ( b mode) and a right mode ( c mode). We also include loss in the mirrors of the cavity as the coupling of the cavity a mode to an additional L mode. These give the following Heisenberg equation of motion for the cavity field, where κ = κ b + κ c + κ L and H sys is the system Hamiltonian (empty cavity or cavity with atom) without considering the baths, which is either Equation (22) can also be written in the equivalent way where k α = κ −2 κ α ; we now consider the output operator for the c mode, wherein the input and output operators are defined as, For the case of an empty cavity, these equations are just a linear system of differential equations and can be solved simply using Fourier transforms defined as to give where These are relations used in the main text when the atom is in the state, as it is assumed to be decoupled from all cavity and environmental modes. However, when the atom is in the state, it is assumed to couple to the cavity a mode. In this situation, one has to include atomic spontaneous emission. This can be done by including the coupling of the transition to an additional bath, E mode, different from the cavity. This gives the set of equations where Г describes the rate of emission into modes other than the cavity modes, and σ in is the input operator of the environment. Note that Г can be made small if the physical cavity mode has a large spatial overlap with the emission pattern of the transition. In the following, we will investigate the system dynamics in the low excitation regime. The reason is twofold. First, we want to avoid exciting the atom in order to prevent decay into the environment (spontaneous emission with the decay rate Г). Second, populating the excited state would induce more complex dynamics, producing in general a nontrivial entangled state between the atom and input, output and cavity fields. This is certainly an interesting regime to investigate in the context of quantum state engineering, but in the present paper we focus on the more intuitive picture in the spirit of (8). The assumption of the atom occupying mostly the ground state can be translated as σ z ≈−. With this assumption, the above set of equations can be solved analytically. Proceeding analogously to the empty cavity case, we have where the unitary matrix with δ a = ω − ω ge , δ c = ω − ω c , s is defined in equation (31), the vector reads and Notice that this set of equations reduces to (30) for the b and c modes, when g =0. Finally, we also assume that all output operators ( b out , c out , L out , E out ) commute with each other, which is not true in general. This approximation is required for an input coherent field in the b in mode to transform into a coherent reflected field in the b out mode and to coherent fields in the c out , L out and E out modes. Finally, as a consistency check of our work, we note that the approximation σ z ≈−1 necessarily requires that the atom remains in the ground state throughout its evolution. Solving for σ ( ω ), one obtains where we have used the fact that the c in and σ in modes represent thermal noise and are thus taken to be negligible compared with the b in mode. Taking the inverse fourier transform, one obtains We then conclude that the self-consistency of our approximation requires that <<1, , which implies that max t P e ( t )<<1. Notice that this condition is a necessary but not sufficient condition for the approximation σ z ≈−1, as this condition itself is derived under the approximation. However, it should be noted that equation (41) can be written in terms of a ( ω ) to obtain Then, for Δ>> ω − ω c , Г, meaning that if the laser addresses only wavelengths close to the bare cavity resonance compared with the detuning between the atom and the cavity, and the atom-cavity detuning is many atomic linewidths away from resonance, one has the condition which is the condition of validity of the dispersive approximation (see Boissonneault et al . [32] ). This means that the condition Δ>> ω − ω c , Г, together with condition max t P e ( t )<<1, is sufficient to justify the approximation σ z ≈−1. Derivation of visibility The state produced after the cavity and beam splitter is of the form where o, b, L and E are the other port of the beam splitter, the reflected field from the cavity, the field loss in cavity mirrors and the spontaneous emission term, respectively. If we measure only the atomic state and the a mode, we lose information in all the other modes. Tracing over the rest of the modes, we obtain the state (9), where visibility, V is, We take only the magnitude of the inner products, as the total phase can, in principle, be compensated by suitable atomic state preparation. This gives the expression where, as in the main text, t BS and r BS are the transmittivity and reflectivity of the beam splitter used in the displacement operation, s L ( ω ) is the spectrum of the laser input field and κ i is the coupling rate of the cavity mode to the i th bath. How to cite this article: Teo, C. et al . Realistic loophole-free Bell test with atom–photon entanglement. Nat. Commun. 4:2104 doi: 10.1038/ncomms3104 (2013). Table 3 Optimized parameters for three points on Fig. 5 Full size table